Regenerable Cu-intercalated MnO2layered cathode for highly cyclable energy dense batteries Manganese dioxide cathodes are inexpensive and have high theoretical capacity (based on two electrons) of 617 mAh g −1 , making them attractive for low-cost, energy-dense batteries. They are used in non-rechargeable batteries with anodes like zinc. Only ∼ 10% of the theoretical capacity is currently accessible in rechargeable alkaline systems. Attempts to access the full capacity using additives have been unsuccessful. We report a class of Bi-birnessite (a layered manganese oxide polymorph mixed with bismuth oxide (Bi 2 O 3 )) cathodes intercalated with Cu 2+ that deliver near-full two-electron capacity reversibly for >6,000 cycles. The key to rechargeability lies in exploiting the redox potentials of Cu to reversibly intercalate into the Bi-birnessite-layered structure during its dissolution and precipitation process for stabilizing and enhancing its charge transfer characteristics. This process holds promise for other applications like catalysis and intercalation of metal ions into layered structures. A large prismatic rechargeable Zn-birnessite cell delivering ∼ 140 Wh l −1 is shown. Batteries for grid applications such as integration of renewable power must be low cost, of high cycle life and energy density, safe, reliable and composed of easily acquired materials requiring relatively simple manufacturing processes [1] . Available technologies for grid applications are often unsuitable for wide deployment because of cost, durability and potential safety hazards [2] , [3] , [4] . High battery energy density is also desirable to minimize installation footprint, for example, for siting in urban areas. Manganese oxide (MnO 2 ) has the desired attributes as an electrode material, being abundant, non-flammable, non-toxic, inexpensive, water-compatible and with a high gravimetric capacity of 617 mAh( g—MnO 2 ) −1 (refs 5 , 6 , 7 , 8 , 9 , 10 , 11 , 12 , 13 , 14 , 15 , 16 , 17 , 18 , 19 , 20 , 21 , 22 , 23 , 24 ). Commonly used primary MnO 2 batteries, where electrolytic manganese dioxide (EMD or γ-MnO 2 ) is paired with zinc (Zn) anodes, have very high-energy densities, >400 Wh l −1 , but can only be discharged once owing to irreversible changes in the γ-MnO 2 crystal structure [13] , [18] , [19] , [20] , [21] , [22] . Limiting the depth of discharge (DOD) to 5–10% of the 617 mAh g −1 MnO 2 gravimetric capacity preserves the reversibility for 1,000–3,000 cycles but reduces energy density to 20 Wh l −1 (ref. 22 ). The low cost of the raw materials makes such low DOD MnO 2 -Zn batteries attractive for grid storage, with costs and cycle life close to the ARPA-E set targets ( http://arpa-e.energy.gov/sites/default/files/documents/files/Volume%201_ARPA-E_ImpactSheetCompilation_FINAL.pdf ). Nonetheless, access of the full second electron capacity of MnO 2 with high cycle life would enable dramatically increased energy density and reduced costs for MnO 2 -Zn batteries. High-energy density batteries for ‘real-world’ applications require electrodes with a combination of high weight percent (wt%) loading of active materials and high areal capacity (mAh cm −2 ), which together would result in high energy density. Unfortunately high wt% loading is often the only parameter reported, which is not the true representation of an energy-dense battery as electrodes can be impractically thin with low active mass per unit area. Among the various polymorphs of manganese dioxide, the birnessite-phase (δ-MnO 2 ) has been known to deliver ∼ 60–80% of the 617 mAh g −1 when cycled at low active mass loadings and under potentiodynamic protocols [15] , [16] , [17] . The rechargeability of the δ-MnO 2 in these prior reports was achieved through additives like Bi 2 O 3 , which mitigated the effects of hausmannite (Mn 3 O 4 ), an electrochemical-inactive phase [15] , [16] , [17] , through [Bi-Mn] complex interactions that maintained the layered structure of birnessite [23] , [24] . However, capacity fade was still an issue, and under galvanostatic cycling protocols, the additives had minimal effect, especially when the wt% loadings or areal capacity of the δ-MnO 2 were high [25] , [26] . The addition of Bi 2 O 3 was useful for low loadings of MnO 2 ; however, at high loadings and galvanostatic cycling, the conductivity of the electrode is crucial, where fast charge transfer characteristics are required [27] . δ-MnO 2 is a very resistive material [28] , and at high loadings, its poor charge transfer characteristics tend to result in the formation of Mn 3 O 4 (ref. 27 ). Prior reports have reported intercalating the δ-MnO 2 -layered structure with ions like cobalt (Co 2+ , Pb 2+ , Ni 2+ ) to improve the electrochemical characteristics for Li-ion batteries [29] , [30] , [31] . However, these intercalants are toxic and/or expensive. In other fields, Cu has been used as an intercalant to improve the properties of layered structures like bismuth selenide [32] , [33] . Cu as an intercalant is attractive in cost and is non-toxic compared to the aforementioned intercalants and it has been shown to improve the electrochemical properties of birnessite [34] , [35] . Here we report the development of Cu 2+ -intercalated layered MnO 2 cathodes with a combination of high wt% loading and high areal capacity (mAh cm −2 ). These cathodes exhibit high volumetric capacity (mAh ml −1 ) and can be regenerated for several thousand charge–discharge cycles delivering nearly the two-electron capacity with minimal capacity fade and at high rate. Cu 2+ intercalated Bi-birnessite (Bi-δ-MnO 2 ) is a layered polymorph of MnO 2 mixed with Bi 2 O 3 and it regenerates via dissolution–precipitation during charge and discharge. The material exploits the redox potential of Cu to intercalate Cu 2+ within the interlayer regions of Bi-δ-MnO 2 during charging, and reduces it as Cu 0 with a Mn(OH) 2 -layered material during discharge. As a consequence, the electrode charge transfer characteristics are greatly improved. This holds promise of dramatically improving energy density and energy storage cost and safety, and amplifies recent interest in birnessite for design of catalysts [36] , lithium (Li) intercalation materials [37] , [38] , [39] and intercalation of metallic ions into layered structures [32] . A large-format rechargeable battery with high loadings of Cu 2+ -intercalated Bi-δ-MnO 2 paired with Zn anodes delivering ∼ 140 Wh l −1 is shown. Electrochemical performance of Bi-δ-MnO 2 with and without Cu Birnessite-layered structure is of resurgent interest for battery applications as an ionic intercalation material [37] , [38] , [39] and with what appears to be some characteristics of a conversion electrode [14] , [15] , [16] , [17] , [27] . Bi-δ-MnO 2 in alkaline electrolyte is synthesized either by an in-situ formation step [15] , [16] , [26] , [40] , [41] by discharging a mix of EMD with Bi 2 O 3 and recharging to its charged state to form Bi-δ-MnO 2 (see Methods section) or by ex situ synthesis methods [14] , [15] , [17] , [23] , [26] , [41] , [42] , [43] , [44] . Both methods have been shown to deliver 60–80% of δ-MnO 2 ’s theoretical capacity (617 mAh g −1 ) at low areal loadings for hundreds of cycles potentiodynamically albeit with constant fade over cycle life [15] , [16] , [17] . Galvanostatically it has been cyclable at low mass loadings with reduced capacity retention [15] , [16] , [17] , [26] . The best results with higher wt% loading from a Bi-δ-MnO 2 cathode were from Kannan et al ., [42] where they showed an ex situ synthesized material could retain ∼ 310–500 mAh g −1 for ∼ 200–600 cycles at C/2 with 50–65 wt% loading. However, there was no mention of areal capacity in the paper and a recent report [44] that used the same synthesis procedure to make Bi-δ-MnO 2 found that at high areal capacity the cycle life was limited to 60 cycles. To the best of our knowledge, there has been no literature data accessing 80–95% of the 617 mAh g −1 of MnO 2 at high mass loadings and areal capacities for thousands of cycles at C rates of interest. To indicate the effects of Cu intercalation on cathode performance, cycling data with and without Cu are presented in Fig. 1 . Cycle one in Fig. 1a shows the material evolution and in situ formation (see Methods section) of Bi-δ-MnO 2 with high areal capacity (21 mAh cm −2 , 45 wt% loading). EMD is mixed with carbon and Bi 2 O 3 and discharged completely to −1 V versus mercury/mercury oxide (Hg/HgO) at C/3 in 37 wt% potassium hydroxide (KOH) solution to form Mn(OH) 2 with Bi. Mn(OH) 2 with Bi is then charged up at C/3 to 0.3 V versus Hg/HgO to form Bi-δ-MnO 2 . Second cycle onwards the flat potential discharge characteristics of the δ-MnO 2 cathode are seen [15] , [16] , [17] ; however, it is not able to retain the capacity. The cause of failure appears to be due to Mn 3 O 4 formation as discussed later in the manuscript. 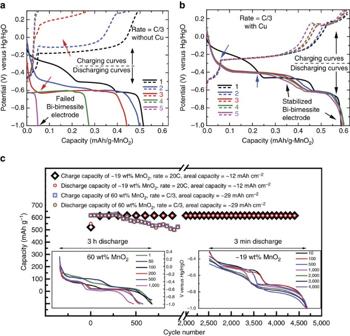Figure 1: Galvanostatic data for Bi-birnessite cathodes with and without Cu additive. (a) First five C/3 cycles of a 45 wt% (∼21 mAh cm−2) EMD, Bi2O3and carbon containing cathode fades completely in five cycles. During the first discharge, potentials characteristic of γ-MnO2were seen. In the second cycle, potentials characteristic of a δ-MnO2layered phase were seen. (b) A comparable electrode with Cu shows negligible capacity fade in five C/3 cycles. (c) Capacity versus cycle number for∼19 and 60 wt% EMD, Bi2O3, Cu and carbon containing cathode at 20C and C/3, respectively. Areal capacities of the∼19 and 60 wt% EMD cells were∼12 and 29 mAh cm−2, respectively, which are indicative of high active loading electrodes. All cycling was against NiOOH counter electrodes. The 60 wt% cell is still cycling at the time of this writing. Figure 1: Galvanostatic data for Bi-birnessite cathodes with and without Cu additive. ( a ) First five C/3 cycles of a 45 wt% ( ∼ 21 mAh cm −2 ) EMD, Bi 2 O 3 and carbon containing cathode fades completely in five cycles. During the first discharge, potentials characteristic of γ-MnO 2 were seen. In the second cycle, potentials characteristic of a δ-MnO 2 layered phase were seen. ( b ) A comparable electrode with Cu shows negligible capacity fade in five C/3 cycles. ( c ) Capacity versus cycle number for ∼ 19 and 60 wt% EMD, Bi 2 O 3 , Cu and carbon containing cathode at 20C and C/3, respectively. Areal capacities of the ∼ 19 and 60 wt% EMD cells were ∼ 12 and 29 mAh cm −2 , respectively, which are indicative of high active loading electrodes. All cycling was against NiOOH counter electrodes. The 60 wt% cell is still cycling at the time of this writing. Full size image Figure 1b shows the cycle performance of a Cu 2+ -intercalated Bi-δ-MnO 2 cathode, which is able to access the theoretical capacity reversibly. The Cu 2+ -intercalated Bi-δ-MnO 2 formation process is very similar, except with the addition of Cu to the mix of EMD, Bi 2 O 3 and carbon. This mix is discharged completely to −1 V versus Hg/HgO and charged to 0.3 V versus Hg/HgO to form Cu 2+ -intercalated Bi-δ-MnO 2 . The effect of Cu is seen, and further cycling reveals that Cu addition is necessary for the stability of Bi-δ-MnO 2 . The discharge potentials (−0.406 V versus Hg/HgO) and charge potentials (−0.26 V versus Hg/HgO) for the Cu-containing electrode (blue arrows) were stable, while those of the electrode without Cu (red arrows) were not. Impedance experiments [45] were performed at the end of charge (0.3 V versus Hg/HgO) for the first five cycles ( Supplementary Fig. 1 ), showing the charge transfer resistance of the Cu-containing electrode to increase from 0.26 to 0.65 mΩ cm −2 , whereas the resistance of the non-Cu electrode increased from 0.78 to 12.7 mΩ cm −2 . High cycling rate (20C) and cycle life (>4,000) of the Cu-intercalated material with a loading of ∼ 19 wt% MnO 2 ( ∼ 12 mAh cm −2 ) is demonstrated in Fig. 1c . The system in general has low charge transfer resistance and can operate at ultrahigh rates. A 60 wt% MnO 2 loading ( ∼ 29 mAh cm −2 ) cell cycled at C/3 is also shown in Fig. 1c , where it is able to access the complete capacity for ∼ 300 cycles, after which it retains >80% of the 617 mAh g −1 over 1,000 cycles. Further, for a series of cells, the wt% loading of EMD was varied from 5 to 45, and the cells were cycled galvanostatically from 1 C to 40 C against nickel oxyhydroxide (NiOOH) counter electrode ( Supplementary Fig. 2 ). The cell performance was stable, delivering a large fraction of the two-electron theoretical capacity. Even at high cycling rates, a high loading cell (45 wt%, ∼ 19 mAh cm −2 ) delivered ∼ 60–65% of the theoretical capacity in galvanostatic cycling at 4C for >1,700 cycles ( Supplementary Fig. 2b ). In several such experiments, much of the capacity was obtained for voltages above −0.6 V, where the effect of the Bi and Cu additives would be expected to contribute little as indicated by the potentiodynamic data in Supplementary Fig. 4 . In some experiments, such as that shown in Supplementary Fig. 2c , the role of the additives on the capacity is more difficult to interpret because some portion of the discharge capacity is extracted at lower voltages. Nonetheless, potentiodynamic data indicate that even in this low voltage region a majority of the capacity is still derived from the MnO 2 ( Supplementary Figs 4 and 5 ). The potentials at which these capacities were obtained appeared to be dependent on wt% loadings and cycling rates. In practical applications, these conditions would need to be optimized. Statistical reliability of the data was also ensured by gathering the average discharge capacity of three similar cells with 50 wt% MnO 2 cycled at 1C, which is shown in Supplementary Fig. 3 , where the standard deviation of the discharged capacity is <2% of the mean. 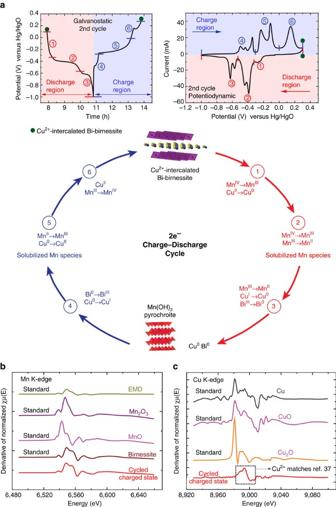Figure 2: Regeneration mechanism and supporting XANES spectra. (a) Electrochemical reactions for the regeneration cycle of Cu2+-intercalated Bi-birnessite. The reactions taking place in each region are colour-coded and numbered corresponding to the galvanostatic and potentiodynamic curves. (b) XANES spectra of a cycled electrode in the charged state for the Mn K edge indicating match with birnessite and (c) for the Cu K-edge of the same material indicating that Cu exists as Cu2+intercalated into birnessite matching ref.37. Regeneration mechanism and electrode characterization Figure 2a shows performance of the second cycle of a Cu 2+ -intercalated Bi-δ-MnO 2 electrode under galvanostatic or potentiodynamic cycling. The slow potentiodynamic cycle (0.1 mV s −1 ) shows the potentials of electrochemical reactions from which the oxidation state of the reactions shown in Fig. 2a were derived. Detailed combinatorial cyclic voltammograms and the reactions are presented in Supplementary Figs 4–6 and Supplementary Table 1 , where each component was methodically added and the electrode potentials were slowly swept to observe the faradaic reactions. The reaction mechanism of Cu 2+ -intercalated Bi-δ-MnO 2 is illustrated in Fig. 2a , wherein three regions of reaction are observered during both charge and discharge. In the discharge region labelled 1, Mn IV and Cu II partially reduce to form Mn III and Cu 0 . The partial reduction of Mn IV is perhaps from surface sites. Discharge region 2 is where Bi-δ-MnO 2 without Cu is previously known to undergo Mn IV to Mn III to Mn II reactions, and here we find that Bi-δ-MnO 2 with Cu also has its significant capacity. This reaction pathway includes a dissolved Mn III state followed by formation of solid Mn(OH) 2 . In the discharge region 3, the remaining Cu I is reduced to Cu 0 and Bi III to Bi 0 . These regions occur for short times and hence the capacity in those regions is small as supported by the low capacity below −0.6 V versus Hg/HgO in Fig. 1b . In the charge region labelled as 4, Bi 0 oxidizes to Bi III with partial oxidation of Cu 0 to Cu I , then substantial charging occurs in region 5 where Mn II is oxidized to Mn III . Just above the dissolution potential of Mn II , Cu 0 also oxidizes to form Cu II , which is present as a dissolved species. In the charge region 6, the formation of Bi-δ-MnO 2 (Mn III to Mn IV ) takes place, and Cu II ions intercalate within the interlayer regions to completely reform Cu 2+ -intercalated Bi-δ-MnO 2 . The mechanism to the improved performance of the Cu 2+ -intercalated Bi-δ-MnO 2 material is that Cu decreases the charge transfer resistance of the δ-MnO 2 , allowing complete regeneration of the materials from the dissolved state during each discharge and charge. Figure 2: Regeneration mechanism and supporting XANES spectra. ( a ) Electrochemical reactions for the regeneration cycle of Cu 2+ -intercalated Bi-birnessite. The reactions taking place in each region are colour-coded and numbered corresponding to the galvanostatic and potentiodynamic curves. ( b ) XANES spectra of a cycled electrode in the charged state for the Mn K edge indicating match with birnessite and ( c ) for the Cu K-edge of the same material indicating that Cu exists as Cu 2+ intercalated into birnessite matching ref. 37 . Full size image Reversible formation of Cu 2+ -intercalated Bi-δ-MnO 2 is confirmed by XANES analysis of an electrode that was cycled 60 times and stopped on charge ( Fig. 2b,c ). The cycled electrode showed characteristic Mn K-edges of a birnessite phase, and also the Cu K-edge matches that of Cu 2+ ions in birnessite [37] , [46] , [47] . The presence of Cu 2+ ions reduces the oxidation state of Mn in Bi-birnessite as seen in Supplementary Fig. 7a . 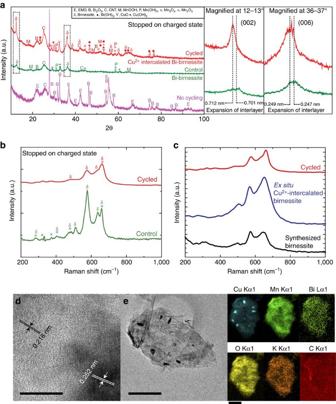Figure 3: Characterization of cycled (with Cu) and control (no Cu) electrodes. (a) XRD of cycled Cu Bi-birnessite, cycled Bi-birnessite without Cu and uncycled initial electrode mix. Magnified panels show interlayer expansion in the case with Cu. (b) Raman spectra of cycled and control electrodes. (c) Raman spectra of cycled electrode, Cu2+-intercalated birnessite producedex situand synthetic birnessite. (d) HRTEM image of the cycled electrode. The darker region and lighter region is indexed to δ-MnO2. (e) TEM EDX mapping of a region of the cycled electrode. Scale bars ind,eare 10 and 500 nm, respectively. Scale bar for maps ineis 250 nm. Figure 3 shows further characterization to confirm the intercalation of Cu 2+ within the layers of birnessite on cycled electrodes (also see Supplementary Figs 7–11 ). Figure 3a shows a X-ray diffraction (XRD) comparison of three materials: a Cu Bi-birnessite electrode cycled 60 times, a control Bi-birnessite electrode with no Cu (failed after four cycles), and non-cycled initial electrode mix. The cycled and control (no-Cu) patterns are both composed predominantly of δ-MnO 2 (indexed to hexagonal space group), indicating the successful Bi-δ-MnO 2 formation process, distinct from the ‘no cyling’ pattern. The c-direction peaks, corresponding to the birnessite interlayer spacing, are shown magnified on the right-side plot. With Cu present, the birnessite interlayer is expanded compared to the control electrode. This expansion is consistent with other reports where metal ions have been intercalated in the birnessite interlayers [31] , [48] . Other peaks are also seen in the XRD of the control electrode, which are indexed to Mn 3 O 4 . To further confirm the fingerprints of these respective phases, Raman spectra was taken for the control and cycled electrode at its charged state. The Raman spectra in Fig. 3b show peaks from the control material match to Mn 3 O 4 (ref. 49 ), whereas different peaks dominate the cycled Cu Bi-δ-MnO 2 material. Raman spectra for synthesized birnessites have the strongest intensity ∼ 575 cm −1 due to the Mn-O stretching along the chains in the MnO 6 sheets followed by a band at ∼ 640–645 cm −1 due to the out of plane stretching of Mn-O in the MnO 6 groups. However, in the Raman spectra of the cycled electrode a significant broadening feature of the band at ∼ 640–645 cm −1 is seen compared to the control electrode. This broadening feature could mean a disruption of the Mn-O caused by the presence of Cu 2+ ions [50] . Ex situ synthetic birnessite was hydrothermally made [51] and soaked in a Cu 2+ solution (copper sulfate (CuSO 4 )) for 48 h, and Raman and XRD were performed. The XRD ( Supplementary Fig. 7c ) for the synthetic Cu-soaked birnessite showed the same peak shifts that were seen in the cycled Cu 2+ -intercalated Bi-birnessite material. The Raman spectra in Fig. 3c also show a match between synthetic birnessite soaked in Cu 2+ and battery-cycled Cu 2+ Bi-δ-MnO 2 , indicating expansion of the birnessite interlayer and pointing the Cu 2+ ions as the origin of the broadening feature [36] , [50] , [52] . This shows that Cu 2+ is intercalated in the Bi-δ-MnO 2 -layered structure during battery cycling, and that this structure is continually reformed upon charging the electrode. Figure 3: Characterization of cycled (with Cu) and control (no Cu) electrodes. ( a ) XRD of cycled Cu Bi-birnessite, cycled Bi-birnessite without Cu and uncycled initial electrode mix. Magnified panels show interlayer expansion in the case with Cu. ( b ) Raman spectra of cycled and control electrodes. ( c ) Raman spectra of cycled electrode, Cu 2+ -intercalated birnessite produced ex situ and synthetic birnessite. ( d ) HRTEM image of the cycled electrode. The darker region and lighter region is indexed to δ-MnO 2 . ( e ) TEM EDX mapping of a region of the cycled electrode. Scale bars in d , e are 10 and 500 nm, respectively. Scale bar for maps in e is 250 nm. Full size image Electron microscopy was also performed to understand the morphological effects of Cu 2+ intercalation. The d-spacing expansion ((0 0 6) direction) from the high-resolution transmission electron microscopy image of the cycled electrode, as shown in Fig. 3d , corroborated the expansion seen in the XRD in Fig. 3a . The energy dispersive X-ray spectroscopy (EDX) mapping image in Fig. 3e and line scan ( Supplementary Fig. 11 ) clearly show the colocation of Cu with Mn throughout the Bi-birnessite nanoparticle, while no Cu was seen in the electrode’s surrounding carbon material. Scanning electron microscopy (SEM) and EDX analysis ( Supplementary Fig. 8a,c ) of the control electrode show an amorphous nature and a Mn to O ratio of ∼ 0.68, indicating Mn 3 O 4 presence. SEM and EDX analysis of the cycled electrodes show sheet-type structures with Cu colocated with Mn ( Supplementary Fig. 8b,d ). EDX of the synthetic, Cu 2+ -soaked birnessite samples showed that Cu 2+ had almost completely replaced the K + ions present within the layers ( Supplementary Fig. 9e–h ). Large-format rechargeable energy-dense cell The in situ synthesis of the δ-MnO 2 using inexpensive, abundant raw materials and the ease of manufacturability make the Cu 2+ -intercalated Bi-δ-MnO 2 an attractive cathode. Ex situ synthesized δ-MnO 2 can also be used with no difference in performance as shown in Supplementary Fig. 12 . From a device standpoint, addition of Cu is not a significant cost contributor because low areal loadings of Cu are sufficient to result in the enhanced capacity and performance ( Supplementary Fig. 13 ). This also indicates that the capacity obtained is predominantly associated with the δ-MnO 2 as the effect of different Cu loadings on capacity is insignificant. We also cycled a Cu cathode against NiOOH counter electrode in a cell of similar design and found that the capacity was <5 mAh g −1 ( Supplementary Fig. 14 ), which supported the finding that Cu added little to the overall capacity of the birnessite cells we tested. To demonstrate the practicality of a Cu 2+ -intercalated Bi-δ-MnO 2 as a battery electrode, in situ synthesized materials were prefered as considerable time and money are saved in comparison to making ex situ synthesized birnessites. The Cu 2+ -intercalated Bi-δ-MnO 2 electrode was cycled against a Zn anode in a large-format prismatic cell with industrial-strength loading of Mn per volume (60 wt%). The battery delivered an energy density of ∼ 160 Wh l −1 for the first cycle and then cycled ∼ 120 Wh l −1 for 90 cycles, as shown in Fig. 4a . This rechargeable aqueous battery possesses a high energy density relative to existing technology, as shown in Fig. 4b . Energy density is currently limited by the Zn DOD (15% in this cell). Zn anodes face cycle life challenges when cycled at more than 10% of theoretical capacity [53] . Calculation shows that when Cu 2+ -intercalated Bi-δ-MnO 2 is paired with a Zn anode that cycles at ∼ 35% of its theoretical capacity, the resulting cell would deliver >250 Wh l −1 , equal to some varieties of Li-ion battery. A comparison of the best MnO 2 cathodes reported in literature is shown in Fig. 4c (see Supplementary Table 2 ), where a striking advancement in cycle life and capacity is noted for Cu 2+ -intercalated Bi-δ-MnO 2 electrodes. An electrode with high areal capacity is preferred as more active mass is used meaning higher energy density and lower cost. 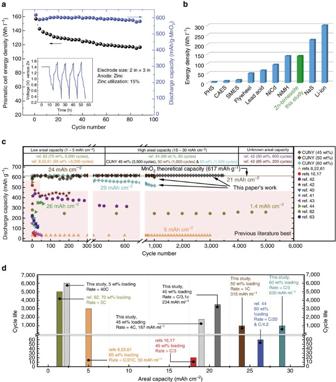Figure 4: Performance characteristics of a Zn-birnessite cell. (a) The discharge energy density (Wh l−1) and capacity (mAh g−1) for a Zn-birnessite cell using the Cu2+-intercalated Bi-birnessite electrode with 60 wt% EMD in the initial mix (continues to cycle at the time of this writing). The voltage-time characteristics for the first 5 cycles are shown in the inset. The electrode sizes are 5.08 cm × 7.62 cm. (b) Energy density comparison of energy storage systems for grid applications59indicating competitive performance of the Cu2+-intercalated Bi-birnessite. (c) Comparison of the best MnO2cathodes reported in literature for aqueous Zn-MnO2batteries. (d) Comparison of the areal capacities and cycle life obtained gathered from reported results in literature60,61,62,63. CAES, compressed air energy storage; PHS, pumped hydro storage; SMES, superconducting magnetic energy storage. Figure 4d illustrates the best areal capacity and cycle life from references in Fig. 4c . Obtaining high cycle life is easy when areal capacities are very low. We show for the first time the attainment of 80–100% of the second electron capacity of MnO 2 with higher areal capacities for thousands of cycles, which also results in high volumetric capacity (mAh ml −1 , see Supplementary Table 2 ). Figure 4: Performance characteristics of a Zn-birnessite cell. ( a ) The discharge energy density (Wh l −1 ) and capacity (mAh g −1 ) for a Zn-birnessite cell using the Cu 2+ -intercalated Bi-birnessite electrode with 60 wt% EMD in the initial mix (continues to cycle at the time of this writing). The voltage-time characteristics for the first 5 cycles are shown in the inset. The electrode sizes are 5.08 cm × 7.62 cm. ( b ) Energy density comparison of energy storage systems for grid applications [59] indicating competitive performance of the Cu 2+ -intercalated Bi-birnessite. ( c ) Comparison of the best MnO 2 cathodes reported in literature for aqueous Zn-MnO 2 batteries. ( d ) Comparison of the areal capacities and cycle life obtained gathered from reported results in literature [60] , [61] , [62] , [63] . CAES, compressed air energy storage; PHS, pumped hydro storage; SMES, superconducting magnetic energy storage. Full size image In conclusion, an MnO 2 cathode with an exceptional combination of reversibility and very high capacity is found to operate via Cu ions intercalated into birnessite-layered structures. The resulting composite material benefits from enhanced charge transfer and complete regeneration of layered materials on each cycle. The application of this methodology is not only limited to batteries but also applies to areas where layered materials are of interest like oxidation catalysts [36] , intercalation chemistry [37] , [38] , [39] and membranes for removal of heavy-metal ions [54] . Materials Manganese sulfate, potassium permanganate and CuSO 4 were purchased from Sigma-Aldrich. Electrolytic manganese dioxide (EMD or γ-MnO 2 , 92%) and bismuth oxide (Bi 2 O 3 , 99.8%) powders were purchased from Tronox Limited and Sigma-Aldrich, respectively. Carboxymethylcellulose sodium (CMC) and polyvinyl alcohol (PVA) were purchased from Sigma-Aldrich. An aqueous binder of 5 wt% CMC-PVA was made by repeated stirring and heating. NiOOH electrodes were purchased from Jiangsu Highstar Battery Manufacturing. Zn (>98%) and zinc oxide (>98%) powders were purchased from Umicore. Teflon was purchased from Dupont. Multiwalled carbon nanotubes (CNTs) were purchased from CNano Technology Limited. Graphite (KS44) was purchased from TIMCAL. KOH pellets were purchased from Fisher Scientific. Synthesis A 6:1 molar solution of potassium permanganate and MnSO 4 was taken in a beaker and mixed till the reactants were completely dissolved. The dissolved solution was kept in a Teflon container and heated at 160 °C for 12 h. The reactants were allowed to cool to room temperature and were finally washed with deionized water three times. The product that was formed was synthetic birnessite. For ex situ intercalation of Cu 2+ , 1 M solution of CuSO 4 was created and mixed with the synthetic birnessite powder for 48 h. The powders were washed with deionized water three times and dried. Electrodes The cathode mix was made by ball milling MnO 2 , Bi 2 O 3 and CNT in appropriate proportions. Slurry was made by adding CMC-PVA and copper (metallic state) to the mix. The mix was pasted onto a nickel mesh, dried and pressed. For the cyclic voltammetry experiments, KS44 was used as the conductive additive. The NiOOH electrodes were commercially made and were used as received. The Zn anodes were made by wet mixing 85% Zn, 10% zinc oxide and 5% Teflon. The mix was then rolled into sheets with a certain thickness and dried at 60 °C for 2 h. The sheets were then cut into appropriate dimensions and pressed onto a copper mesh [55] , [56] . The utilization of the Zn was 15%. Cell assembly The electrodes were assembled into a prismatic box (2.54 cm depth × 8.26 cm width × 21.6 cm height) made of polysulfone. The inner diameter of the polysulfone box where the electrodes are compressed is 1.94 cm. Cellophane was used as the separator in the cells that contained NiOOH as the counter electrode. The NiOOH electrodes were sealed in polyolefin nonwoven membrane (FS 2192SG; Freudenberg). The cathodes were wrapped with three layers of cellophane and then paired with two NiOOH electrodes and uniformly compressed in the prismatic box with polypropylene shims. The electrode sizes tested in this cell assembly were 2.54 cm × 2.54 cm and 5.08 cm × 7.62 cm, respectively. In the Zn-birnessite cell, the electrodes were fitted in the above polysulfone box as well. The cathode was wrapped in three layers of cellophane, and the Zn anode was sealed in polyolefin nonwoven membrane (FS 2192SG; Freudenberg) and Celgard 5550 (Celgard). A pack consists of one cathode and anode with the aforementioned separators was compressed in the prismatic box with polypropylene shims. The pack’s total thickness of 0.163 cm consists of 0.046 cm cathode, 0.058 cm anode, 0.013 cm cellophane, 0.030 cm FS 2192SG and 0.015 cm Celgard 5550. A volume of 0.0063 L is calculated from the electrode area (5.08 cm × 7.62 cm) times the pack thickness. Electrochemical tests The impedance experiments (EIS) were performed on 5.08 cm × 7.62 cm electrodes. NiOOH electrodes were used as the counter electrode. The cathodes used in the tests had 45 wt% with the balance being covered by Bi 2 O 3 , CNT and CMC-PVA for the Bi-birnessite electrode, and the same mix with Cu for the Cu 2+ -intercalated Bi-birnessite. The EIS was performed at a frequency range of 20 kHz to 0.1 Hz at an AC amplitude of 5 mV. The cyclic voltammetry experiments were performed on a 2.54 cm × 2.54 cm electrode. NiOOH electrodes were used as the counter electrode. The cathodes used in the tests had 5 wt% active material loading of MnO 2 with the remaining balance covered by Bi 2 O 3 , Cu, KS44 and CMC-PVA. In the tests where there was no MnO 2 , the main active material was Bi 2 O 3 . The weight ratio of KS-44 to active material was ∼ 17. 37 wt%. KOH was used as the electrolyte. A Hg/HgO reference electrode was used to monitor the cathode. The tests were run at 0.1 mV s −1 between 0.3 and −1 V against the reference. The tests were conducted on a Biologic potentiostat/galvanostat (VSP Modular 5-channel) instrument. The galvanostatic experiments were performed on a 2.54 cm × 2.54 cm and 5.08 cm × 7.62 cm electrodes. NiOOH or Zn was used as the counter electrodes. The cathode had 45–60 wt% loading of MnO 2 with the balance being covered by Bi 2 O 3 , Cu, CNT and CMC-PVA. The 60 wt% MnO 2 loading electrode did not contain any CMC-PVA. The molar ratio of Bi 2 O 3 to MnO 2 was around 0.04 irrespective of MnO 2 loading percentages. For the 10 C and 20 C tests, around 19 wt% loading of MnO 2 was used, and for the 40 C test, around 5 wt% MnO 2 loading was used. KOH of 25 wt% was used for the Zn anodes and 37 wt% of KOH was used for the NiOOH counter electrodes. A Hg/HgO reference electrode was used in the tests where NiOOH was the counter electrode. The tests were run at C/3 against Zn, and at C/3, 1 C, 4 C, 10 C, 20 C and 40 C in the cells with NiOOH as the counter electrode. All the capacity calculations are based on the mass of MnO 2 used in the mix. The cell cycling protocols were set to access the 617 mAh g −1 (theoretical limit of MnO 2 ) between 0.3 and −1 V versus Hg/HgO. The galvanostatic tests were carried out on a multichannel Arbin BT 2000. In situ synthesis of Bi-birnessite Cycle one (black curves) in Fig. 1a shows the electrochemical in situ formation process of Bi-δ-MnO 2 against a NiOOH counter electrode. EMD (45 wt%) is mixed with carbon powder and Bi 2 O 3 and discharged completely (to −1 V versus Hg/HgO, black solid curve) at C/3 in 37 wt% KOH solution to form Mn(OH) 2 . The sigmoidal part ( ∼ −0.15 to −0.5 V versus Hg/HgO) of the solid black curve indicates the proton (H + ) intercalation process into the tunnel structure of EMD to form MnOOH. This represents the first electron reaction, which delivers ∼ 308 mAh g −1 . The flat part of the solid black curves ( ∼ −0.5 to −1 V versus Hg/HgO) represents the second electron reaction (delivering ∼ 308 mAh g −1 ), where the dissolution–precipitation of the Mn ions [57] , [58] from MnOOH to form Mn(OH) 2 and Bi 2 O 3 reduction to form Bi metal (see Supplementary Table 1 ) takes place. The discharged product (Mn(OH) 2 with Bi) is then charged up at C/3 to birnessite’s formation potentials (0.3 V versus Hg/HgO; Supplementary Table 1 has detailed reactions) to finally form Bi-δ-MnO 2 . The Bi 2 O 3 role in this process is to maintain the layered structure through [Bi-Mn] interactions [32] , [33] , which are seen in the peaks of potentiodynamic cycling ( Fig. 2 ) and to a lesser extent in the galvanostatic curves of Fig. 1a . Second cycle onwards the flat potential discharge characteristics (solid blue, red, green and pink curves) of the Bi-δ-MnO 2 cathode are seen. The Cu 2+ intercalated Bi-δ-MnO 2 is formed through the same in situ formation step, except with the addition of Cu to the mix of EMD, Bi 2 O 3 and carbon. Material characterization XRD and Raman spectroscopy were performed on all the materials. The materials were also viewed under an SEM and a TEM. XRD was carried out on a PANalytical X’Pert Pro Powder Diffraction instrument fitted with a PIXcel 1D fast detector and Cu Kα filter. Raman measurements were taken on a MonoVista Confocal Raman Microscope with SP 2750 series spectrograph from Princeton Instruments-Action and an upright Olympus BX51 confocal microscope. SEM images were taken on a Zeiss Supra 55 VP field emission microscopy fitted with an EDX. TEM images were taken on a JEOL JEM2100 microscope fitted with an Inca EDX system, and also with STEM (scanning transmission electron microscopy) capabilities. Gold grids were used for the TEM and EDX analyses. XANES was taken on the 5-ID (SRX) beamline of the National Synchrotron Light Source II at Brookhaven National Laboratory, New York. Multiple measurements were taken for different MnO 2 and copper standards. For the Mn K-edge, EMD, MnO, Mn 2 O 3 and synthesized birnessite were used for the Mn standards. For the Cu K-edge, metallic Cu, CuO and Cu 2 O were used for the Cu standards. All the XANES data was analysed in Athena. The characterization work was performed on ex situ samples, which were washed and dried in their charged states, which could have resulted in some oxidation, perhaps explaining the minor peak of CuO in the XRD. Data availability The authors declare that the data supporting the findings of this study are available from the corresponding author on reasonable request. How to cite this article: Yadav, G. G. et al . Regenerable Cu-intercalated MnO 2 layered cathode for highly cyclable energy dense batteries. Nat. Commun. 8, 14424 doi: 10.1038/ncomms14424 (2017). Publisher’s note : Springer Nature remains neutral with regard to jurisdictional claims in published maps and institutional affiliations.